Significant performance enhancement in photoconductive terahertz optoelectronics by incorporating plasmonic contact electrodes Even though the terahertz spectrum is well suited for chemical identification, material characterization, biological sensing and medical imaging, practical development of these applications has been hindered by attributes of existing terahertz optoelectronics. Here we demonstrate that the use of plasmonic contact electrodes can significantly mitigate the low-quantum efficiency performance of photoconductive terahertz optoelectronics. The use of plasmonic contact electrodes offers nanoscale carrier transport path lengths for the majority of photocarriers, increasing the number of collected photocarriers in a subpicosecond timescale and, thus, enhancing the optical-to-terahertz conversion efficiency of photoconductive terahertz emitters and the detection sensitivity of photoconductive terahertz detectors. We experimentally demonstrate 50 times higher terahertz radiation powers from a plasmonic photoconductive emitter in comparison with a similar photoconductive emitter with non-plasmonic contact electrodes, as well as 30 times higher terahertz detection sensitivities from a plasmonic photoconductive detector in comparison with a similar photoconductive detector with non-plasmonic contact electrodes. There has been a great deal of effort for extending the high-frequency limit of radio frequency (RF) sources and the low-frequency limit of optical emitters, as well as combining RF and optical techniques to realize high-performance terahertz radiation sources [1] . On the RF side, impact ionization avalanche transit-time diodes, Gunn diodes, resonance tunneling diodes and chains of frequency multipliers [2] , [3] , [4] have demonstrated very promising compact terahertz sources. However, this category of sources has limited bandwidth, poor power efficiency and low output power levels. On the other hand, electron beam devices such as backward wave oscillators [5] and travelling wave tube regenerative amplifiers [6] can produce reasonable power levels, but their operation has not been demonstrated above 1.5 THz (ref. 7 ). Additionally, the bulky nature of backward wave oscillators and their requirement for high magnetic fields and vacuum limit their use in various operational settings. On the optical side, quantum-cascade lasers have been under an extensive investigation during the past decade [8] , and significant progress has been made, pushing their operation frequency to 1 THz (ref. 9 ) and their operation temperature to ~200 K for a 3.22-THz lasing frequency [10] . Moreover, optical down-conversion to terahertz frequencies based on nonlinear optical effects has been extensively used for generating high-power terahertz waves. Optical down-conversion to terahertz frequencies in bulk nonlinear materials is inherently inefficient due to the optical/terahertz phase mismatch limiting the efficient field interaction length. Guided wave nonlinear media [11] , quasi-phase-matching in periodically poled media [12] , [13] and the use of tilted wave-front pump waves [14] have been used to offer a better phase-matching control, resulting in longer field interaction lengths. However, because of material absorption, the active length in which terahertz waves are generated is limited to centimetre ranges. Because of the field interaction length limitations, the use of high-power optical pumps has been necessary to provide ultra-high peak powers for generating meaningful terahertz powers using nonlinear optical techniques. An additional inherent limitation of nonlinear optical techniques for generating terahertz waves stems from the conservation of energy in a nonlinear optical process, namely the Manley–Rowe rule [15] . In other words, the maximum power efficiency of terahertz sources based on nonlinear optical phenomena is limited to the ratio between the energies of the generated terahertz photon and the pump optical photon. On the other hand, optical-to-terahertz conversion through photoconduction has demonstrated very promising performance [16] , [17] , [18] , [19] , [20] , [21] , [22] and has been the most commonly used technique for generating terahertz waves since the pioneering demonstration of picosecond photoconducting Hertzian dipoles in 1984 (ref. 23 ). One of the main advantages of photoconductive terahertz emitters compared with the terahertz emitters based on nonlinear optical phenomena is that their power efficiency is not restricted by the Manley–Rowe limit. This is because one electron-hole pair can be generated for each absorbing photon, which can emit several terahertz photons on reaching the terahertz antenna in a photoconductive emitter. In other words, the optical-to-terahertz conversion efficiency of photoconductive terahertz emitters can reach 100%, orders of magnitude higher than the Manley–Rowe limit. Although the optical-to-terahertz conversion efficiency of photoconductive emitters can theoretically reach 100%, the low-quantum efficiency of conventional ultrafast photoconductors imposes substantially lower conversion efficiencies. The low-quantum efficiency of conventional ultrafast photoconductors also limits the responsivity and detection sensitivity of photoconductive terahertz detectors, which are extensively used in combination with photoconductive terahertz emitters in time-domain and frequency-domain terahertz spectroscopy and imaging systems [24] , [25] . To address the low-quantum efficiency limitation of conventional ultrafast photoconductors, we propose a novel photoconductor concept that incorporates a plasmonic contact electrode configuration to offer high quantum efficiency and ultrafast operation simultaneously. By using nanoscale plasmonic contact electrodes we significantly reduce the average photocarrier transport path to the photoconductor contact electrodes compared with conventional photoconductors. By incorporating plasmonic contact electrodes, we demonstrate enhancing the optical-to-terahertz power conversion efficiency of a conventional photoconductive terahertz emitter by a factor of 50. By use of the same quantum efficiency enhancement mechanism, we also demonstrate increase in the responsivity and detection sensitivity of a conventional photoconductive terahertz detector by a factor of 30. Consequently, our presented plasmonic photoconductive terahertz optoelectronics concept offers more than three orders of magnitude enhancement in the signal-to-noise ratio of time-domain and frequency-domain terahertz spectroscopy and imaging systems. Plasmonic photoconductors for terahertz generation To demonstrate the potential of plasmonic electrodes for enhancing the quantum efficiency of conventional ultrafast photoconductors, we chose to fabricate a proof-of-concept photoconductive emitter and characterize its performance enhancement due to integrating plasmonic gratings as a part of photoconductor contact electrodes. 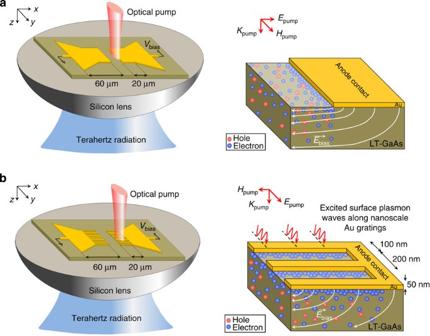Figure 1: Schematic diagram and operation concept of photoconductive terahertz emitters and detectors. Left panels: an ultrafast photoconductor connected to a bowtie terahertz antenna on a LT-GaAs substrate. The device is mounted on a silicon lens to collect the terahertz radiation from back side of the substrate. An optical pump is incident on the ultrafast photoconductor, generating electron-hole pairs inside the photo-absorbing substrate. Right panels: to operate as a terahertz emitter, a bias voltage is applied to the ultrafast photoconductor, which induces an electric field inside the substrate and drifts the photo-generated electrons and holes towards the anode and cathode contact electrodes, respectively. On reaching the contact electrodes, the photocurrent drives the terahertz antenna to produce radiation. To operate as a terahertz detector, a zero bias voltage is applied to the ultrafast photoconductor, and the bowtie terahertz antenna connected to the contact electrodes of the ultrafast photoconductor receives the incident terahertz radiation, inducing a terahertz electric field across the photoconductor contact electrodes. The photo-generated electrons and holes are drifted to the photoconductor contact electrodes under the induced terahertz field, generating an output photocurrent that is proportional to the magnitude of the incident terahertz field. (a) A conventional photoconductive terahertz emitter/detector. (b) A plasmonic photoconductive terahertz emitter/detector incorporating plasmonic contact electrodes to reduce photocarrier transport times to the contact electrodes and, thus, increase the photoconductor quantum efficiency. Figure 1a shows the schematic diagram and operation concept of the implemented photoconductive emitter in the absence of plasmonic gratings (conventional scheme). The photoconductive emitter consists of an ultrafast photoconductor with 20 μm gap between the anode and cathode contacts, connected to a 60-μm-long bowtie antenna with maximum and minimum widths of 100 and 30 μm, respectively. Low-temperature-grown GaAs (LT-GaAs) is used for the photo-absorbing substrate to achieve an ultrafast photoconductor response. When a subpicosecond optical pump at ~800 nm wavelength range is incident on the ultrafast photoconductor, electron-hole pairs are generated that induce a photocurrent under an applied bias electric field. The induced photocurrent, which follows the envelope of the optical pump, drives the terahertz antenna connected to the photoconductor contact electrodes, generating terahertz radiation. The bandwidth of the terahertz radiation is determined by the optical pulse, antenna characteristics and the semiconductor carrier lifetime. As electrons have significantly higher mobilities compared with holes and due to the nonlinear increase in the bias electric field near the contact electrodes, the optical pump is focused onto the photoconductive gap asymmetrically close to the anode contact to maximize terahertz radiation [19] , [26] , [27] . Similar to any conventional photoconductive terahertz emitter, the quantum efficiency of the described photoconductive emitter is limited by the relatively long carrier transport path lengths to the photoconductor contact electrodes. This is because of the relatively low drift velocity of the carriers in the semiconductor [28] , and even if the pump is focused down to a diffraction-limited spot size next to the anode contact, a very small portion of the photo-generated electrons can reach the anode in a subpicosecond timescale. The remaining majority of the photo-generated carriers recombine in the substrate before reaching the contact electrodes and without efficient contribution to terahertz generation. Figure 1b shows the schematic diagram of the implemented photoconductive emitter that incorporates 20-μm-long plasmonic contact electrode gratings designed for enhancing the quantum efficiency of the conventional photoconductive emitter ( Fig. 1a ). The grating geometry is designed to excite surface plasmon waves along the periodic metallic grating interface on incidence of a transverse magnetic-polarized optical pump [29] , [30] . Excitation of surface plasmon waves allows transmission of a large portion of the optical pump through the nanoscale grating into the photo-absorbing substrate. It also significantly enhances the intensity of the optical pump in very close proximity to the contact electrodes. As a result, the average photo-generated electron transport path length to the anode electrode is significantly reduced in comparison with the conventional photoconductive emitter ( Fig. 1a ). Therefore, the design strategy for the optimum plasmonic grating is maximizing the optical pump transmission into the photo-absorbing substrate while minimizing the electrode spacing to minimize the average photo-generated electron transport path length to the anode electrode. Figure 1: Schematic diagram and operation concept of photoconductive terahertz emitters and detectors. Left panels: an ultrafast photoconductor connected to a bowtie terahertz antenna on a LT-GaAs substrate. The device is mounted on a silicon lens to collect the terahertz radiation from back side of the substrate. An optical pump is incident on the ultrafast photoconductor, generating electron-hole pairs inside the photo-absorbing substrate. Right panels: to operate as a terahertz emitter, a bias voltage is applied to the ultrafast photoconductor, which induces an electric field inside the substrate and drifts the photo-generated electrons and holes towards the anode and cathode contact electrodes, respectively. On reaching the contact electrodes, the photocurrent drives the terahertz antenna to produce radiation. To operate as a terahertz detector, a zero bias voltage is applied to the ultrafast photoconductor, and the bowtie terahertz antenna connected to the contact electrodes of the ultrafast photoconductor receives the incident terahertz radiation, inducing a terahertz electric field across the photoconductor contact electrodes. The photo-generated electrons and holes are drifted to the photoconductor contact electrodes under the induced terahertz field, generating an output photocurrent that is proportional to the magnitude of the incident terahertz field. ( a ) A conventional photoconductive terahertz emitter/detector. ( b ) A plasmonic photoconductive terahertz emitter/detector incorporating plasmonic contact electrodes to reduce photocarrier transport times to the contact electrodes and, thus, increase the photoconductor quantum efficiency. Full size image Incorporating a dielectric passivation layer could reduce the Fresnel reflection at the semiconductor interface and, thus, could enhance optical pump transmission into the photo-absorbing semiconductor for both conventional and plasmonic photoconductors [31] , [32] . While optical pump transmission into the photo-absorbing semiconductor of the conventional photoconductor is the result of direct interaction between the pump wave and the semiconductor interface, optical pump transmission into the photo-absorbing semiconductor of the plasmonic photoconductor is through coupling to the excited surface plasmon waves. Because of the differences between the nature of the interacting waves with the semiconductor interface, the optimum passivation layer thicknesses, which maximize optical pump transmission into the photo-absorbing semiconductor, are not the same for the conventional and plasmonic photoconductors. While the passivation layer thickness can be independently optimized for each photoconductor, we have chosen the passivation layer thicknesses to obtain the same optical pump transmission into the photo-absorbing semiconductor for the conventional and plasmonic photoconductors. We used a 150-nm SiO 2 passivation layer for the plasmonic photoconductor with Au contact gratings having a 200 nm pitch, 100 nm spacing and 50 nm height and no passivation layer for the conventional photoconductor. Both designs offer ~70% optical pump transmission into the photo-absorbing semiconductor at a 800-nm optical pump wavelength ( Supplementary Fig. S1 ). Using a multi-physics finite-element solver (COMSOL), we have analysed the interaction of an incident optical pump ( λ =800 nm) with the conventional and plasmonic photoconductors. For maximum optical power enhancement near the photoconductor contact electrodes, we have aligned the optical pump field along the x axis and y axis for the conventional and plasmonic photoconductors, respectively [33] . The optical absorption in the semiconductor substrate for the conventional ( xz cross-section) and plasmonic ( yz cross-section) photoconductors is shown in Fig. 2a. For the conventional photoconductor, the metal contact shadows the substrate from the incident optical pump, allowing for almost all of the optical absorption and photocarrier generation in the gap between the anode and cathode. In the case of the plasmonic photoconductor, the optical pump is transmitted through the nanoscale metallic grating through the coupling with surface plasmons. As the excited surface plasmon waves exist at the dielectric-metal interface, the highest optical absorption and photocarrier generation occurs in direct proximity to the metal contacts. To better illustrate the impact of the excited surface plasmon waves, we have compared the optical absorption profile in the semiconductor substrate of the photoconductor with nanoscale Au gratings with a similar photoconductor with nanoscale Ni gratings. 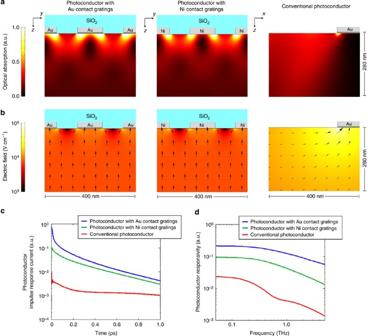Figure 2: Finite element analysis of optical and electrical interactions in the photoconductor cross-sections. Right panel: cross-section of the conventional photoconductor (xz-plane). Left and centre panels: cross-sections of the designed plasmonic photoconductor and a similar photoconductor with Ni contact gratings (yz-plane). A 5-nm-thick Ti adhesion layer is deposited under Au electrodes. A 150-nm-thick SiO2passivation layer is used for the photoconductors with nanoscale contact gratings and no passivation layer is used for the conventional photoconductor. This allows equal optical transmission to the photo-absorbing substrate (~70%) at 800 nm optical pump wavelength for all three photoconductors. (a) Colour plot of optical absorption in GaAs substrate due to an incident optical plane wave (λ=800 nm). The optical pump field is aligned along thexaxis andyaxis for the conventional photoconductor and photoconductors with nanoscale contact gratings, respectively. (b) Bias electric field in GaAs substrate. Colour map corresponds to electric field magnitude, and arrows denote field direction. Applied voltages in all three cases are set to not exceed electric fields of 1 × 105V cm−1. The cross-sections of the photoconductors with nanoscale contact gratings are shown for a distance 1 μm inset from the tip of the gratings. (c) Estimated impulse response of the analysed photoconductors with the illustrated cross-sections by combining the photo-generated carrier density in the GaAs substrate, the electric field data and the classical drift-diffusion model in a multi-physics finite-element solver (COMSOL) and calculating the induced photocurrent in response to an optical pump impulse. A carrier lifetime of 400 fs is assumed for the LT-GaAs substrate. (d) Estimated responsivity spectra of the analysed photoconductors calculated by convolving the impulse response of each photoconductor with the sinusoidal power envelope of two frequency-offset optical beams as a function of optical beat frequency. a.u., arbitrary unit. Figure 2a shows that under the same optical transmission through nanoscale Au and Ni gratings, the highest optical absorption and photocarrier generation regions are more tightly confined at the metal-semiconductor interface of Au gratings in comparison with Ni gratings. This is explained by the weak plasmonic properties of Ni at 800-nm optical wavelength. Using COMSOL, we have analysed the bias electric field that drifts photo-generated carriers towards the photoconductor contact electrodes ( Fig. 2b ). For this analysis, the bias voltage is set such that the maximum induced electric field remains below 10 5 V cm −1 (1/4th of the GaAs breakdown electric field). In the case of the conventional photoconductor, we see elliptical electric field lines beneath the contact electrode with the highest electric field near the corner of the electrodes. In the case of the plasmonic photoconductor, the electric field lines are illustrated at the yz cross-section 1 μm away from the grating tip. Although relatively lower electric fields are induced in the case of the plasmonic photoconductor compared with the conventional photoconductor, the electric field levels are maintained above 10 3 V cm −1 (at which electron drift velocity reaches saturation) within 100 nm from photoconductor anode contact electrodes [28] . Moreover, simulation results show that the electric field levels are maintained above 10 3 V cm −1 within 100 nm from contact electrodes along a 20-μm-long plasmonic contact electrode, indicating that the superior performance of the plasmonic photoconductive emitter can be maintained when using relatively large device active areas. Figure 2: Finite element analysis of optical and electrical interactions in the photoconductor cross-sections. Right panel: cross-section of the conventional photoconductor ( xz -plane). Left and centre panels: cross-sections of the designed plasmonic photoconductor and a similar photoconductor with Ni contact gratings ( yz -plane). A 5-nm-thick Ti adhesion layer is deposited under Au electrodes. A 150-nm-thick SiO 2 passivation layer is used for the photoconductors with nanoscale contact gratings and no passivation layer is used for the conventional photoconductor. This allows equal optical transmission to the photo-absorbing substrate (~70%) at 800 nm optical pump wavelength for all three photoconductors. ( a ) Colour plot of optical absorption in GaAs substrate due to an incident optical plane wave ( λ =800 nm). The optical pump field is aligned along the x axis and y axis for the conventional photoconductor and photoconductors with nanoscale contact gratings, respectively. ( b ) Bias electric field in GaAs substrate. Colour map corresponds to electric field magnitude, and arrows denote field direction. Applied voltages in all three cases are set to not exceed electric fields of 1 × 10 5 V cm −1 . The cross-sections of the photoconductors with nanoscale contact gratings are shown for a distance 1 μm inset from the tip of the gratings. ( c ) Estimated impulse response of the analysed photoconductors with the illustrated cross-sections by combining the photo-generated carrier density in the GaAs substrate, the electric field data and the classical drift-diffusion model in a multi-physics finite-element solver (COMSOL) and calculating the induced photocurrent in response to an optical pump impulse. A carrier lifetime of 400 fs is assumed for the LT-GaAs substrate. ( d ) Estimated responsivity spectra of the analysed photoconductors calculated by convolving the impulse response of each photoconductor with the sinusoidal power envelope of two frequency-offset optical beams as a function of optical beat frequency. a.u., arbitrary unit. Full size image The impulse response of the analysed photoconductors to an optical pump impulse is estimated by calculating the collected transient photocurrent at the contact electrodes using COMSOL. For this purpose, the photo-generated carrier density is derived from the calculated optical intensity in the GaAs substrate and combined with the electric field data in the classical drift-diffusion model to calculate the induced photocurrent. The results are presented in Fig. 2c, indicating the superior performance of the designed plasmonic photoconductor offering high-quantum efficiency and ultrafast operation simultaneously. The advantage of the designed plasmonic photoconductor is more apparent when comparing its responsivity with the conventional photoconductor and the photoconductor with Ni contact gratings. The responsivity spectra are calculated by convolving the impulse response of the analysed photoconductors with the sinusoidal power envelope of two frequency-offset optical beams as a function of optical beat frequency. The responsivity spectra ( Fig. 2d ) show that the designed plasmonic photoconductor offers more than one order of magnitude higher responsivity levels compared with the conventional photoconductor. Moreover, comparing the responsivity spectra of the designed plasmonic photoconductor with the photoconductor with Ni contact gratings indicates the impact of plasmonic optical enhancement in direct proximity to the metal contacts, which offers higher photoconductor responsivity levels, especially at higher terahertz frequencies. It should be mentioned that at a given pump power, the radiated power from a photoconductive emitter has a quadratic dependence on the photoconductor responsivity. Therefore, compared with the conventional photoconductor, the designed plasmonic photoconductor is expected to offer two orders of magnitude higher optical-to-terahertz conversion efficiencies. 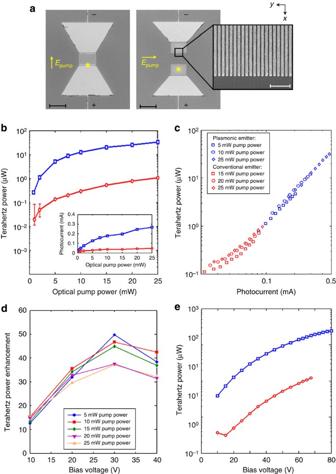Figure 3: Comparison of the conventional and plasmonic photoconductive terahertz emitter prototypes. (a) Fabricated device images. Left: microscope image of the conventional terahertz emitter with a 20 μm scale bar. Middle: microscope image of the plasmonic terahertz emitter with a 20 μm scale bar. Right: scanning electron microscopy image of the plasmonic electrodes of the plasmonic terahertz emitter with a 1 μm scale bar. The circular pump spot is positioned on the antenna axis at the anode contact edge and along the anode plasmonic contact electrodes for the conventional and plasmonic photoconductive emitters, respectively. (b) Measured terahertz radiation from the plasmonic (blue) and conventional (red) terahertz emitters, electrically biased at 40 V, under various optical pump powers. The inset curve shows the corresponding photocurrent of the plasmonic (blue) and conventional (red) emitters. The error bars are associated with the noise of the pyroelectric terahertz detector listed in the detector datasheet. (c) Measured terahertz radiation versus collected photocurrent for the plasmonic and conventional terahertz emitters. The data represented in the plot includes various bias voltages (10–40 V) under various optical pump powers (5–25 mW). (d) Relative terahertz power enhancement defined as the ratio of the terahertz power emitted by the plasmonic terahertz emitter to the conventional terahertz emitter. Maximum enhancement is obtained at low optical powers before the onset of the carrier screening effect. (e) Maximum terahertz power measured from the plasmonic (blue) and conventional (red) terahertz emitters under a 100 mW optical pump. The bias voltage of each device is increased until the point of device failure. a.u., arbitrary unit. Figure 3a shows the microscope and scanning electron microscopy images of the fabricated photoconductive emitter prototypes. Figure 3: Comparison of the conventional and plasmonic photoconductive terahertz emitter prototypes. ( a ) Fabricated device images. Left: microscope image of the conventional terahertz emitter with a 20 μm scale bar. Middle: microscope image of the plasmonic terahertz emitter with a 20 μm scale bar. Right: scanning electron microscopy image of the plasmonic electrodes of the plasmonic terahertz emitter with a 1 μm scale bar. The circular pump spot is positioned on the antenna axis at the anode contact edge and along the anode plasmonic contact electrodes for the conventional and plasmonic photoconductive emitters, respectively. ( b ) Measured terahertz radiation from the plasmonic (blue) and conventional (red) terahertz emitters, electrically biased at 40 V, under various optical pump powers. The inset curve shows the corresponding photocurrent of the plasmonic (blue) and conventional (red) emitters. The error bars are associated with the noise of the pyroelectric terahertz detector listed in the detector datasheet. ( c ) Measured terahertz radiation versus collected photocurrent for the plasmonic and conventional terahertz emitters. The data represented in the plot includes various bias voltages (10–40 V) under various optical pump powers (5–25 mW). ( d ) Relative terahertz power enhancement defined as the ratio of the terahertz power emitted by the plasmonic terahertz emitter to the conventional terahertz emitter. Maximum enhancement is obtained at low optical powers before the onset of the carrier screening effect. ( e ) Maximum terahertz power measured from the plasmonic (blue) and conventional (red) terahertz emitters under a 100 mW optical pump. The bias voltage of each device is increased until the point of device failure. a.u., arbitrary unit. Full size image Fabrication began with the patterning of the nanoscale gratings using electron beam lithography, followed by Ti/Au (5/45 nm) deposition and liftoff to form ohmic photoconductor contacts ( Supplementary Fig. S2 ) [34] . A 150-nm-thick SiO 2 passivation layer was then deposited using plasma-enhanced chemical vapor deposition (PECVD). Using a plasma etcher, contact vias were then opened, and the antenna and metal contacts were formed using optical lithography followed by Ti/Au (5/400 nm) deposition and liftoff. The fabricated devices were then mounted on a silicon lens and placed on an optical rotation mount, for optical pump polarization adjustments. To evaluate the performance of the photoconductive terahertz emitter with and without the plasmonic gratings, the output power of each device was measured in response to an incident optical pump from a Ti:sapphire mode-locked laser with a central wavelength of 800 nm, 76 MHz repetition rate and 200 fs pulse width, using a pyroelectric detector (Spectrum Detector Inc., SPI-A-65 THz). To maximize terahertz radiation, the incident optical pump was tightly focused onto each device and the circular pump spot was positioned on the antenna axis at the anode contact edge and along the anode plasmonic contact electrodes for the conventional and plasmonic photoconductive emitters, respectively, as illustrated in Fig. 3a ( Supplementary Fig. S3a ). Moreover, the device rotation mount was adjusted to align the electric field of the optical pump along the x axis and y axis for the conventional and plasmonic prototypes, respectively ( Supplementary Fig. S3b ). The measured output power of the two prototype devices at a 40-V bias voltage and under various optical pump powers is presented in Fig. 3b. A radiation power enhancement of more than 33 was observed from the plasmonic photoconductive emitter in the 0–25 mW optical pump power range. This significant radiation power enhancement is due to the higher photocurrent levels generated when employing plasmonic contact electrodes ( Fig. 3b inset), which have a quadratic relation with the radiation power. Another important advantage of the plasmonic emitter compared with the conventional emitter is that the close photocarrier proximity to contact electrodes is satisfied over significantly larger device active areas and, thus, the operation of the plasmonic emitter is more immune from optical pump misalignment. While the radiated power from the conventional emitter decreases dramatically as a result of optical pump displacement along the x axis, the plasmonic emitter does not show any noticeable decrease in power as a result of the optical pump displacement along the 20-μm-long anode plasmonic contact electrodes. To further examine the impact of photocurrent increase on the radiation power enhancement, we compared the radiation power of the two photoconductor devices as a function of their photocurrent under various bias voltages (10–40 V) and optical pump powers (5–25 mW). The results are presented in Fig. 3c in a logarithmic scale. The data points are all curve-fitted to the same line with a slope of 2, confirming the quadratic dependence of the radiation power on the induced photocurrent and the fact that all other operational conditions (including antenna specifications) are the same for the conventional and plasmonic photoconductive emitter prototypes. By dividing the output power of the plasmonic photoconductive emitter by the output power of the conventional photoconductive emitter, we define a power enhancement factor. Figure 3d shows the power enhancement factor under various optical pump powers and bias voltages. At low optical pump power levels and a bias voltage of 30 V, output power enhancement factors up to 50 are observed, the same order of magnitude predicted by the theoretical predictions. The enhancement factor decreases slightly at higher optical pump power levels. This can be explained by the carrier screening effect, which affects the plasmonic photoconductor more than the conventional photoconductor, as a larger number of electron-hole pairs are separated in the plasmonic photoconductor. Additionally, the enhancement factor decreases slightly at higher bias voltages. This is because stronger forces separate electron-hole pairs at higher bias voltages. As a larger number of electron-hole pairs contribute to the induced photocurrent in the plasmonic photoconductor compared with the conventional photoconductor, the relative increase in the induced electric field opposing the bias electric field, as a function of the bias electric field, is higher in the plasmonic photoconductor. It should be also mentioned that the lower enhancement factors at bias voltages below 30 V are associated with insufficient bias electric field levels along the plasmonic contact electrodes of the plasmonic photoconductor. Finally, the maximum radiated power from each photoconductive terahertz emitter was measured at an optical pump power of 100 mW, up to the point that the devices burned, as shown in Fig. 3e. At maximum, the plasmonic photoconductive emitter produced an average power of 250 μW, compared with the 12 μW of the conventional photoconductive emitter. The time-domain ( Fig. 4a ) and frequency-domain ( Fig. 4b ) radiation of the plasmonic photoconductive emitter in response to a 200-fs optical pump pulse from the Ti:sapphire mode-locked laser was measured using a terahertz time-domain spectroscopy setup with electro-optic detection [25] . The detailed description of the terahertz time-domain spectroscopy setup used for characterizing the photoconductive terahertz emitter prototypes can be found in the Methods section. The radiated power from the plasmonic terahertz source was detected up to 1.5 THz, after which the noise of the system limited the detection. The observed radiation peaks around 0.35 and 0.55 THz are associated with the resonance peaks of the employed bowtie antenna, and the radiation peak around 0.1 THz is associated with the resonance peak of the dipole antenna formed by the bowtie antenna bias lines. 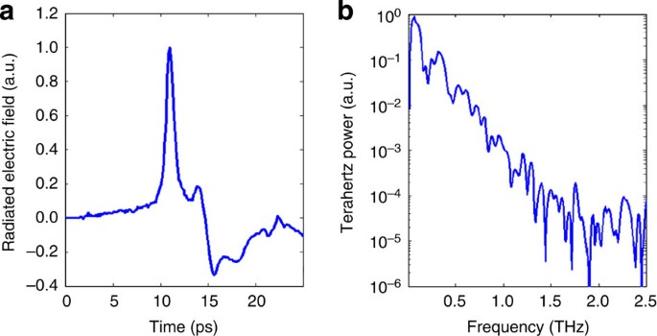Figure 4: Radiation characteristics of the plasmonic photoconductive emitter. (a) Radiated electric field in the time domain in response to a 200-fs optical pulse from the Ti:sapphire mode-locked laser with 800 nm central wavelength and 76 MHz repetition rate. (b) Radiated power in the frequency domain, obtained by calculating the Fourier transform of the measured time-domain terahertz electric field intensity. a.u., arbitrary unit. Figure 4: Radiation characteristics of the plasmonic photoconductive emitter. ( a ) Radiated electric field in the time domain in response to a 200-fs optical pulse from the Ti:sapphire mode-locked laser with 800 nm central wavelength and 76 MHz repetition rate. ( b ) Radiated power in the frequency domain, obtained by calculating the Fourier transform of the measured time-domain terahertz electric field intensity. a.u., arbitrary unit. Full size image Plasmonic photoconductors for terahertz detection Following the demonstration of terahertz radiation enhancement by use of plasmonic contact electrodes, we evaluated the potential of plasmonic electrodes for enhancing the detection sensitivity of conventional photoconductive terahertz detectors by characterizing the performance of the fabricated proof-of-concept photoconductors in terahertz detection mode. Figure 1a shows the schematic diagram and operation concept of the proof-of-concept photoconductive terahertz detector in the absence of the plasmonic gratings (conventional scheme). Photocarriers are generated inside the active area of the ultrafast photoconductor on incidence of an optical pump. The terahertz antenna connected to the contact electrodes of the ultrafast photoconductor receives the incident terahertz radiation and induces a terahertz electric field across the photoconductor contact electrodes. The induced terahertz field drifts the photocarriers towards the photoconductor contact electrodes, generating an output photocurrent that is proportional to the magnitude of the incident terahertz field. The responsivity of the conventional photoconductive terahertz detector is directly affected by the number of the photocarriers that reach the photoconductor contact electrodes within a subpicosecond timescale. Similar to the conventional photoconductive terahertz emitter, the quantum efficiency of the described conventional photoconductive terahertz detector is limited by the relatively long carrier transport path lengths to the photoconductor contact electrodes. Therefore, even if the optical pump is focused down to a diffraction-limited spot size next to the photoconductor contact electrodes, a small portion of the photocarriers can reach the photoconductor contact electrodes within a subpicosecond timescale, limiting the responsivity of the conventional photoconductive terahertz detector. Figure 1b shows the schematic diagram of the proof-of-concept photoconductive terahertz detector that incorporates plasmonic contact electrode gratings (plasmonic scheme). Similar to the plasmonic photoconductive terahertz emitter, the use of plasmonic contact electrodes reduces the average transport path of the photocarriers to the photoconductor contact electrodes considerably. This results in a significant increase in the number of the drifted photocarriers to the photoconductor contact electrodes and, thus, the output photocurrent of the plasmonic photoconductive detector in comparison with the conventional photoconductive detector under the same incident terahertz wave intensities. To evaluate the performance of the photoconductive terahertz detector with and without the plasmonic gratings, the output photocurrent of each device in response to the radiation from a commercially available photoconductive terahertz emitter (iPCA-21-05-1000-800-h) was measured in a time-domain terahertz spectroscopy setup. The detailed description of the terahertz time-domain spectroscopy setup used for characterizing the photoconductive terahertz detector prototypes can be found in the Methods section. A Ti:sapphire mode-locked laser with a central wavelength of 800 nm, 76 MHz repetition rate and 200 fs pulse width was used for pumping the commercially available photoconductive terahertz emitter and the photoconductive terahertz detector prototypes in the terahertz time-domain spectroscopy setup. The optical pump polarization was set along the x axis and y axis for the conventional and plasmonic photoconductive detectors, respectively, and both photoconductive detector prototypes were characterized under the same optical pump and terahertz radiation intensities. To achieve the highest output photocurrent levels from the photoconductive detector prototypes, the optical pump was tightly focused onto each device and the circular pump spot was asymmetrically positioned onto the photoconductive gap of each device. To have a fair comparison between the performance of the conventional and plasmonic photoconductive terahertz detectors, each measurement was repeated for various optical pump spot positions along the photoconductive gap until the highest output photocurrent level is achieved for each detector prototype ( Fig. 5 ). The measured time-domain output photocurrent of the conventional and plasmonic photoconductive terahertz detectors is shown in Fig. 5a. While the output photocurrent of both photoconductive detectors follow the envelope of the received electric field from the photoconductive terahertz emitter used in the terahertz spectroscopy setup, 30 times higher output photocurrent levels are offered by the plasmonic photoconductive terahertz detector. Additionally, the calculated frequency components of the measured time-domain output photocurrents ( Fig. 5b ) indicate that the 30-fold output photocurrent enhancement offered by the plasmonic photoconductive terahertz detector is maintained over a 0.1–1.5 THz frequency band. The output noise level of the conventional and plasmonic photoconductive detector prototypes is estimated by measuring the time-domain output photocurrent of each photoconductive detector while blocking the incident terahertz radiation, and subsequently calculating the frequency components of the measured time-domain output photocurrents. The results indicate similar output noise current spectra for the conventional and plasmonic photoconductive detector prototypes ( Supplementary Fig. S4a ). This is due to the fact that the dominant noise source in both photoconductive detectors is the Johnson–Nyquist noise rather than the photoconductor shot noise ( Supplementary Fig. S4b,c ). Therefore, the 30-fold responsivity enhancement offered by the plasmonic photoconductive detector enables achieving 30 times higher detection sensitivities over the 0.1–1.5 THz frequency band. 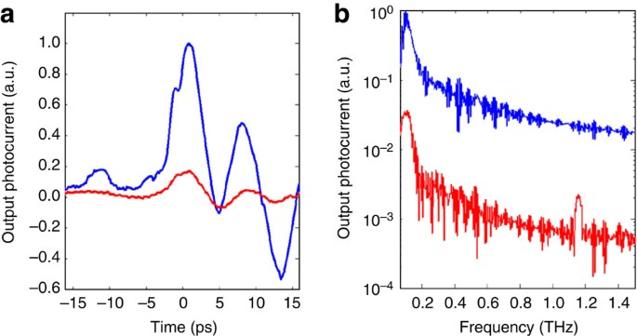Figure 5: Comparison of the conventional and plasmonic photoconductive terahertz detector prototypes. (a) Time-domain output photocurrent of the conventional photoconductive terahertz detector × 5 (red) and plasmonic photoconductive terahertz detector × 1 (blue), measured in a time-domain terahertz spectroscopy setup under an optical pump power of 50 mW. While the output photocurrent of both photoconductive detectors follow the envelope of the received electric field from the photoconductive terahertz emitter used in the terahertz spectroscopy setup, 30 times higher responsivity levels are offered by the plasmonic photoconductive terahertz detector. (b) Frequency-domain output photocurrent of the conventional (red) and plasmonic (blue) photoconductive terahertz detectors, obtained by calculating the Fourier transform of the measured time-domain output photocurrents. The calculated frequency components of the measured output photocurrents indicate that the 30-fold responsivity enhancement offered by the plasmonic photoconductive terahertz detector is maintained over a 0.1–1.5 THz frequency band. a.u., arbitrary unit. Figure 5: Comparison of the conventional and plasmonic photoconductive terahertz detector prototypes. ( a ) Time-domain output photocurrent of the conventional photoconductive terahertz detector × 5 (red) and plasmonic photoconductive terahertz detector × 1 (blue), measured in a time-domain terahertz spectroscopy setup under an optical pump power of 50 mW. While the output photocurrent of both photoconductive detectors follow the envelope of the received electric field from the photoconductive terahertz emitter used in the terahertz spectroscopy setup, 30 times higher responsivity levels are offered by the plasmonic photoconductive terahertz detector. ( b ) Frequency-domain output photocurrent of the conventional (red) and plasmonic (blue) photoconductive terahertz detectors, obtained by calculating the Fourier transform of the measured time-domain output photocurrents. The calculated frequency components of the measured output photocurrents indicate that the 30-fold responsivity enhancement offered by the plasmonic photoconductive terahertz detector is maintained over a 0.1–1.5 THz frequency band. a.u., arbitrary unit. Full size image The ability to excite surface plasmon waves has enabled many unique opportunities for routing and manipulating electromagnetic waves [35] . It has enabled strong light concentration in the near-field, paving the way for higher resolution imaging and spectroscopy [36] , [37] , deep electromagnetic focusing and beam shaping [38] , [39] , higher efficiency photovoltaics [40] , [41] , photodetectors [42] , [43] , modulators [44] , [45] and photoconductors [22] . On the basis of this capability, we have proposed and experimentally demonstrated 50 times radiation power enhancement and 30 times detection sensitivity enhancement by incorporating plasmonic contact electrodes in a photoconductive terahertz emitter and detector, respectively. Subsequently, the presented plasmonic photoconductive terahertz optoelectronics concept enhances the signal-to-noise ratio of conventional time-domain and frequency-domain terahertz spectroscopy and imaging systems by more than three orders of magnitude. Plasmonic electrodes are designed to significantly reduce the average carrier transport distance to photoconductor contact electrodes over relatively large device active areas and without a considerable increase in the capacitive loading to the terahertz radiating antenna. This enables boosting the maximum terahertz radiation power and detection sensitivity [46] , [47] , [48] , [49] , [50] , [51] by mitigating the carrier screening effect [52] , semiconductor bleaching [53] and thermal breakdown [54] at high optical pump powers. It should be noted that the focus of this study has been the demonstration of the impact of plasmonic electrodes in enhancing the quantum efficiency of ultrafast photoconductors and, thus, the radiation power and detection sensitivity of photoconductive terahertz emitters and detectors, respectively. Hence the choice of the photoconductive emitter/detector architecture, terahertz radiating/receiving antenna and bias feed in our study has been arbitrary, and the enhancement concept can be similarly applied to enhance the performance of photoconductive terahertz emitters/detectors with a variety of terahertz antennas with and without interdigitated contact electrodes as well as large-area photoconductive terahertz emitters/detectors in both pulsed and continuous-wave operation. In this regard, the output power and detection sensitivity of our prototype devices can be further enhanced through use of resonance cavities [26] , [29] and antennas with higher radiation resistance and bandwidth [55] , [56] . Moreover, the use of high aspect ratio plasmonic contact electrodes embedded inside the photo-absorbing semiconductor [57] , [58] allows a larger number of carriers generated in close proximity with photoconductor contact electrodes and, thus, enables further terahertz radiation power and detection sensitivity enhancement. In this regard, extending the plasmonic electrode height to dimensions larger than the optical pump absorption depth allows ultrafast transport of the majority of photocarriers to the photoconductor contact electrodes and their efficient contribution to terahertz generation and detection. This eliminates the need for using short carrier lifetime semiconductors, which are used for suppressing the DC current of photoconductive emitters/detectors (in general) and for preventing undesired destructive interferences in continuous-wave photoconductive emitters/detectors (specifically) [59] . Eliminating the need for using short carrier lifetime semiconductors, which have lower carrier mobilities and thermal conductivities [54] compared with high-quality crystalline semiconductors, would have an important impact on future high efficiency photoconductive terahertz emitters and detectors. Spectral characterization of terahertz emitters The terahertz radiation of the photoconductive terahertz emitter prototypes is monitored in time-domain and frequency-domain through a terahertz time-domain spectroscopy setup with electro-optic detection. The beam from a Ti:sapphire mode-locked laser with a central wavelength of 800 nm, 76 MHz repetition rate and 200 fs pulse width is split into a pump beam and a probe beam. The pump beam is modulated by an optical chopper and focused onto the device under test. The emitted radiation is collimated and subsequently focused using two polyethylene spherical lenses in the ambient atmosphere. Before the focal point of the second polyethylene lens, the terahertz radiation is combined with the optical probe beam using an indium tin oxide (ITO)-coated glass filter. Both paths are then focused onto a 1-mm thick, <110> ZnTe crystal. The terahertz electric field is measured indirectly by monitoring the polarization state of the probe beam. This is accomplished by setting the optical probe polarization at a 45° angle relative to the terahertz polarization before the ZnTe crystal (by use of a half-waveplate) and converting the optical probe polarization into a circular polarization after the ZnTe crystal (by use of a quarter-waveplate), followed by a Wollaston prism to split the circularly polarized optical probe beam into two branches. The power of the two output beams from the Wollaston prism is measured by two balanced photodetectors connected to a lock-in amplifier with the optical pump modulation reference. By inserting a controllable optical delay line in the optical probe path, the time delay between the optical probe and terahertz pulses interacting inside the ZnTe crystal is varied, and the time-domain terahertz electric field is measured accordingly. The frequency-domain radiation of the photoconductive terahertz emitter prototypes is obtained by calculating the Fourier transform of the measured time-domain terahertz electric field intensity. Spectral characterization of terahertz detectors The performance of the photoconductive terahertz detector prototypes is characterized in a time-domain terahertz spectroscopy setup with photoconductive detection. The beam from a Ti:sapphire mode-locked laser with a central wavelength of 800 nm, 76 MHz repetition rate and 200 fs pulse width is split into a pump beam and a probe beam. The pump beam is focused onto a commercially available photoconductive terahertz emitter (iPCA-21-05-1000-800-h) and the emitted radiation is modulated by controlling the bias voltage of the photoconductive terahertz emitter. The emitted radiation is collimated and subsequently focused onto the photoconductive terahertz detector prototypes under test, using two polyethylene spherical lenses in the ambient atmosphere. The probe beam is used for pumping the photoconductive terahertz detector prototypes under test. The output current of the photoconductive terahertz detector prototypes is measured by a lock-in amplifier with the optical probe modulation reference. By inserting a controllable optical delay line in the optical pump path, the time delay between the optical probe and terahertz pulses is varied, and the time-domain output photocurrent of the photoconductive terahertz detector prototypes is measured accordingly. The frequency-domain output photocurrent of the photoconductive terahertz detector prototypes is obtained by calculating the Fourier transform of the measured time-domain output photocurrent. How to cite this article: Berry, C. W. et al . Significant performance enhancement in photoconductive terahertz optoelectronics by incorporating plasmonic contact electrodes. Nat. Commun. 4:1622 doi: 10.1038/ncomms2638 (2013).